Photoinitiated charge separation in a hybrid titanium dioxide metalloporphyrin peptide material In natural systems, electron flow is mediated by proteins that spatially organize donor and acceptor molecules with great precision. Achieving this guided, directional flow of information is a desirable feature in photovoltaic media. Here, we design self-assembled peptide materials that organize multiple electronic components capable of performing photoinduced charge separation. Two peptides, c16-AHL 3 K 3 -CO 2 H and c16-AHL 3 K 9 -CO 2 H, self-assemble into fibres and provide a scaffold capable of binding a metalloporphyrin via histidine axial ligation and mineralize titanium dioxide (TiO 2 ) on the lysine-rich surface of the resulting fibrous structures. Electron paramagnetic resonance studies of this self-assembled material under continuous light excitation demonstrate charge separation induced by excitation of the metalloporphyrin and mediated by the peptide assembly structure. This approach to dye-sensitized semiconducting materials offers a means to spatially control the dye molecule with respect to the semiconducting material through careful, strategic peptide design. The flow of energy and information in natural systems is governed by carefully positioned donor and acceptor molecules [1] . The electrons flow through bond, through space or via a hopping mechanism. Developing a functional material that controls the flow of electrons based on these principles of nature is prevalent but often implementation of structural elements is lost. The conformation and relative spatial separation between the two components dictates the efficiency and the rate at which electrons are transferred. The protein serves as the architectural scaffold for organizing the molecules which, in turn, provides its ultimate function. For example, the well-known intensely green coloured molecule chlorophyll is an excellent light-harvesting molecule but really offers very little utility when functioning alone. When the protein light-harvesting complex II found in purple bacteria binds and organizes the chromophore, the required light-harvesting properties for initiating the transformation of light into food are achieved [2] , [3] . This is but one example of nature’s achievement in employing proteins to govern the flow of electrons. The elegance of photoinduced charge separation, as found in nature, inspired the design for dye-sensitized solar cells (DSCs) [4] , [5] . In a DSC, a porous network of crystalline titanium(IV) dioxide (TiO 2 ) nanoparticles, is sensitized by the random adsorption or coordination of a dye molecule to the surface of the semiconducting metal oxide particles. On illumination, the dye molecule injects an electron into the conduction band of TiO 2 resulting in efficient charge separation. To date, the record conversion efficiency was achieved with a zinc metalloporphyrin dye, η eff =12.7% (ref. 6 ). Significant loss in efficiency is possibly due to the multiple electron and energy transfer pathways after the initial photoexcitation process. Although it is difficult to compare the efficiencies of photovoltaic devices to natural photosynthetic systems where the overall efficiency is often cited as an optimistic 3%, much of the energy loss that occurs is nature’s intent for reasons of regeneration, environment and many other factors that are problems relevant to systems biology [7] , [8] , [9] . Nature is therefore purposely directing its electrons through guided pathways utilizing the harvested light in multiple processes. Therefore, developing a material that can control the direction of electron flow based on natural principles will provide necessary insight towards the importance of structural arrangement in a photovoltaic medium. Here, we take inspiration from the same natural source that resulted in DSCs, light-harvesting systems [2] , [3] , [10] . Much of the current work for varying the distance and orientation of the dye molecule relative to the surface of the semiconducting material relies extensively on the synthesis of new dye molecules [11] , [12] , [13] , [14] . We have developed an alternative, strategic approach to organizing the dye molecule and the semiconducting material by employing a self-assembled peptide amphiphile as the structural template. The design has been shown to bind and organize a variety of metalloporphyrins on extensive length scales in the form of fibrillar structures [15] . The resulting structure produces a surface rich in lysine residues, which have been shown to induce TiO 2 mineralization by both unassembled and assembled peptide systems in good yield [16] , [17] , [18] , [19] , [20] , [21] . The final material is a peptide fibre that internally binds a metalloporphyrin and externally mineralizes TiO 2 . As the dye molecule is not attached to the semiconducting particle through a covalent bridge, the pathway for electron transfer occurs either through space or the peptide. The present work highlights our ability to generate a complex material from simple starting precursors that is capable of non-covalently organizing donor and acceptor moieties such that the material yields a charge-separated state upon illumination with visible light. Design The use of novel architectures in photovoltaic and photocatalytic systems stems from the influence of nature that employs guided pathways for electron transfer. The ultimate goal is to have a simple design guided by natural principles that yields a complex structure that dictates donor and acceptor organization. Here, we combine a peptide, a synthetic metalloporphyrin (5,15-diphenylporphyrin)Zinc, (DPP)Zn, and titania precursor, Fig. 1 , that self-assemble into an architecture capable of photoinduced charge transfer, Fig. 2 . The peptides were designed as described before [15] . Briefly, an aliphatic c16 tail was incorporated to induce hydrophobic collapse. A moderate β-sheet foldamer [22] , [23] , [24] made up of three leucine residues was used to provide a handle on the formation of the fibre-like structure. The histidine was placed towards the interior, nonpolar region of the peptide to allow for axial coordination of the water insoluble (DPP)Zn. And the exterior lysines produce a highly positively charged region that when neutralized at high pH, induces β-sheet formation and fibre formation. The lysine-rich exterior is then capable of mineralizing TiO 2 on the assembled peptide’s surface yielding the complex hybrid material, Fig. 2 . Two peptides c16-AHL 3 K 3 -CO 2 H and c16-AHL 3 K 9 -CO 2 H were produced to observe the dependence of mineralization on the number of lysine residues present. The peptides were synthesized by standard Fmoc based solid-phase synthesis and purified by reversed phase high-performance liquid chromatography. The identity of the peptides was confirmed by matrix-assisted laser desorption/ionization–mass spectrometry. 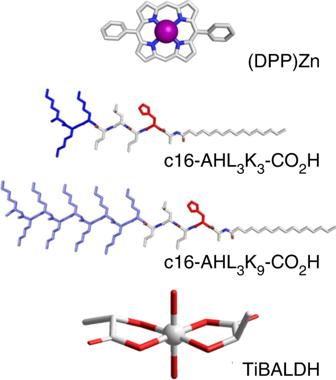Figure 1: Precursor molecules for the metalloporphyrin/metal oxide arrays. . Figure 1: Precursor molecules for the metalloporphyrin/metal oxide arrays. . 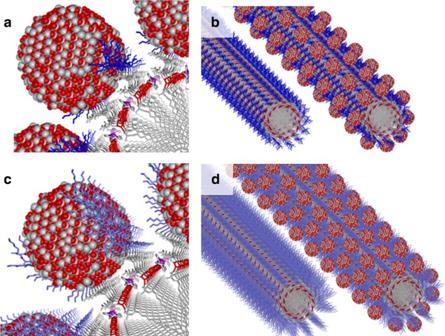Figure 2: Self-assembled peptide/(DPP)Zn/TiO2arrays. (a) Detail of the interface and (b) cartoon depiction of the self-assembled morphology for c16-AHL3K3-CO2H/(DPP)Zn/TiO2and analogous depictions (c,d) for c16-AHL3K9-CO2H/(DPP)Zn/TiO2. Full size image Figure 2: Self-assembled peptide/(DPP)Zn/TiO 2 arrays. ( a ) Detail of the interface and ( b ) cartoon depiction of the self-assembled morphology for c16-AHL 3 K 3 -CO 2 H/(DPP)Zn/TiO 2 and analogous depictions ( c , d ) for c16-AHL 3 K 9 -CO 2 H/(DPP)Zn/TiO 2 . Full size image Peptide assembly The self-assembled peptide amphiphile material was generated under slightly altered conditions from our previous report, namely the samples were heated to induce β-sheet formation. Briefly, a 250 μM solution of the peptide amphiphile was made by mixing a portion of a fluid 1 wt% solution of the peptide into 100 mM ammonium hydroxide, then heated to 65 °C for 10 min. The peptides self-assemble into nanofibers via neutralization of the lysine residues (pKa~10.5) which trigger β-sheet assembly and the propagation of nanofiber formation. c16-AHL 3 K 3 -CO 2 H assembles into bundled fibres as previously reported. The unusual circular dichroism spectrum λ min =229 nm is red shifted from the β-sheet signature spectrum λ min =218 nm and was previously established to be a result of twisted and/or aggregated bundles of β-sheet containing nanofibers, see Supplementary Fig. 1 (ref. 15 , 25 , 26 ). This is consistent with the electron microscopy image detailing the very long and bundled features of the assembled material, see Supplementary Fig. 2 . Interestingly, c16-AHL 3 K 9 -CO 2 H assembles into less-bundled nanofibers. This is most likely due to the significant increase in lysine residues yielding greater electrostatic repulsion between neighbouring fibres. When c16-AHL 3 K 9 -CO 2 H in 100 mM ammonium hydroxide is heated to 65 °C and then cooled back to room temperature (RT), CD yields a spectrum slightly red shifted from a typical β-sheet spectrum, λ min =224 nm, see Supplementary Fig. 1 (refs 25 , 26 ). Electron microscopy shows nanoscale bundled fibres, see Supplementary Fig. 3 . This observation is consistent with the supposition correlating the CD data with the microscopy data in that the more red-shifted spectra indicate a higher degree to which the fibres are twisted and aggregated. To understand this difference in assembly between the two peptides, thermal assembly studies were executed in which the n-π* bands of the circular dichroism spectrum were monitored, λ mon =210 and 222 nm, while varying the temperature from 10–65 °C, see Supplementary Fig. 1 . The data indicates a greater enthalpic barrier to β-sheet formation in the case of c16-AHL 3 K 9 -CO 2 H ( T m =48 °C) when compared with c16-AHL 3 K 3 -CO 2 H ( T m =28 °C). The presence of the additional lysine residues clearly contributes to this barrier. Mineralization Mineralization of inorganic materials by organisms is a natural phenomenon observed in the formation of shells, spines and fibres in protists, diatoms and sponges; and bone in mammals [27] , [28] , [29] . These structures are all induced by peptide sequences with specific characteristics. For example, a high isoelectric point is a common characteristic of peptides and proteins that yield metal-oxides [16] , [17] , [18] , [19] , [20] . One well-studied example is the water soluble titania precursor, Titanium(IV) bis-ammonium lactato dihydroxy (TiBALDH), which can be converted to TiO 2 in the presence of peptides rich in lysine and arginine [16] , [17] , [18] . The mechanism of mineralization is often attributed to an initial electrostatic interaction between the negatively charged titania precursor and the positively charged lysine residues which effectively creates locally concentrated areas of titania. This is followed by dissociation of the lactato ligands and subsequent hydrolysis of the vacant reaction site on the titania [30] . As a result, TiO 2 is formed. This observation has yielded a peptide design guideline for interfacing peptides with TiO 2 such that peptides exhibiting exposed lysine and/or arginine residues possess the mineralization property. It has also been reported that mineralization of metal oxides on self-assembled peptide surfaces can dictate the morphology of the inorganic material [21] , [31] . To that effect, the peptides discussed here, c16-AHL 3 K 3 -CO 2 H and c16-AHL 3 K 9 -CO 2 H, are excellent candidates for exploring TiO 2 mineralization. Two conditions were examined, the disassembled peptide in water and the assembled peptide in ammonium hydroxide solutions. The peptides were diluted from a fluid 1 wt% stock solution in water to a 500 μM solution in water or ammonium hydroxide and heated to 65 °C. After allowing the samples to cool to RT, TiBALDH was added to each sample to achieve a 1 wt% (35 mM) solution. The unassembled samples immediately became turbid indicative of mineralization, whereas the assembled samples did not show immediate turbidity. All samples were heated to 65 °C for 10 min to ensure completion of the mineralization reaction. The samples were washed by pelleting via centrifugation, removal of the supernatant followed by resuspension with the respective solvents three times. Note: control samples were made in the absence of peptide under identical conditions to ensure that TiO 2 formation was not a result of thermal degradation. The morphology of the material was analysed by scanning electron microscopy equipped with a transmission detector. The samples in water exhibited clusters of TiO 2 in no discernible assembly, Fig. 3a,d . Samples prepared in ammonium hydroxide exhibited maintenance of the nanofibre structures, but decorated in TiO 2 nanoparticles (<3 nm), Fig. 3b,e . Particles were specifically observed on the assembled peptide surface. The presence of titania was confirmed via EDX spectroscopy and energy-filtered transmission electron microscopy (EFTEM), see Supplementary Fig. 4 . The two peptides were employed under the supposition that c16-AHL 3 K 9 -CO 2 H would produce either larger particles or more particles than c16-AHL 3 K 3 -CO 2 H. Not only does c16-AHL 3 K 9 -CO 2 H have a longer poly-lysine chain, but it also yields extensive individual fibres as observed in the electron microscopy in the absence of TiO 2 , see Supplementary Fig. 3 . This provides a greater exposed lysine surface area. By electron microscopy, we find that indeed c16-AHL 3 K 9 -CO 2 H yields more particles on the peptide surface than c16-AHL 3 K 3 -CO 2 H, see Supplementary Fig. 5 (TEM). In the case of c16-AHL 3 K 9 -CO 2 H, smaller fibres and bundles of fibres were observed suggesting that the addition of TiBALDH does not promote the bundling of fibres. The presence of TiO 2 yields a higher contrast producing noticeably different images, see Supplementary Figs 3 and 3e . For c16-AHL 3 K 3 -CO 2 H, the observed bundling remains in both the presence and absence of TiO 2 . Although, it appears that the fibres become more rigid and brittle in the presence of TiO 2 . 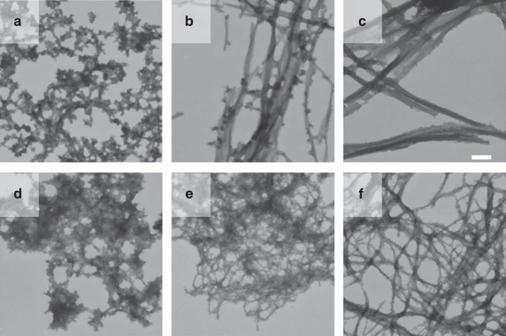Figure 3: Mineralization of TiO2on unassembled and assembled peptide amphiphiles. Electron micrographs of mineralized TiO2on (a) unassembled c16-AHL3K3-CO2H, (b) assembled c16-AHL3K3-CO2H, (c) with (DPP)Zn, (d) unassembled c16-AHL3K9-CO2H, (e) assembled c16-AHL3K9-CO2H and (f) with (DPP)Zn. Scale bar, 200 nm for all images. Figure 3: Mineralization of TiO 2 on unassembled and assembled peptide amphiphiles. Electron micrographs of mineralized TiO 2 on ( a ) unassembled c16-AHL 3 K 3 -CO 2 H, ( b ) assembled c16-AHL 3 K 3 -CO 2 H, ( c ) with (DPP)Zn, ( d ) unassembled c16-AHL 3 K 9 -CO 2 H, ( e ) assembled c16-AHL 3 K 9 -CO 2 H and ( f ) with (DPP)Zn. Scale bar, 200 nm for all images. Full size image By employing high resolution transmission electron microscopy (HRTEM), we were able to determine that the mineralized TiO 2 was crystalline, Fig. 4 , and indexing of the electron diffraction pattern indicated an anatase crystal phase, see Supplementary Fig. 6 . The quantity of crystalline particles on c16-AHL 3 K 9 -CO 2 H exceeds that of c16-AHL 3 K 3 -CO 2 H. One unusual aspect observed in the bundles of fibres of the two peptide assemblies is that c16-AHL 3 K 3 -CO 2 H, which features more rigid fibres appeared to organize the particles in between neighbouring bundles yielding some organization to the particles on the fibres whereas c16-AHL 3 K 9 -CO 2 H yielded densely packed yet entangled fibres, see Supplementary Fig. 5 (TEM). These two observations provide a potentially useful platform when examining the interplay between self-assembly and particle assembly and its effects on the particles’ collective properties. 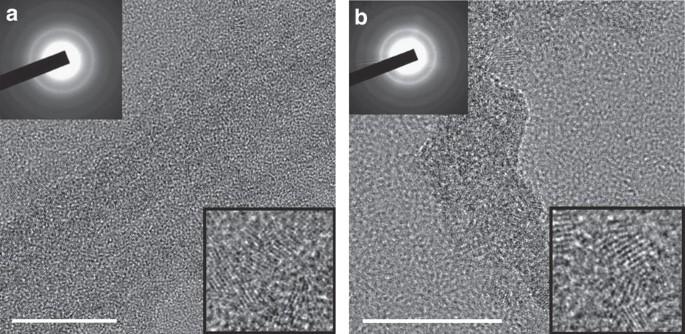Figure 4: Evidence of anatase formed at ambient temperatures. HRTEM micrograph of mineralized nanocrystalline TiO2on the surface of self-assembled peptides (a) c16-AHL3K3-CO2H and (b) c16-AHL3K9-CO2H. Insets: Electron diffraction and magnified view of observed crystal lattices. Scale bar, 20 nm for both images. Figure 4: Evidence of anatase formed at ambient temperatures. HRTEM micrograph of mineralized nanocrystalline TiO 2 on the surface of self-assembled peptides ( a ) c16-AHL 3 K 3 -CO 2 H and ( b ) c16-AHL 3 K 9 -CO 2 H. Insets: Electron diffraction and magnified view of observed crystal lattices. Scale bar, 20 nm for both images. Full size image Quantification of TiO 2 While the electron microscopy indicates a greater population of particles on the assembled c16-AHL 3 K 9 -CO 2 H peptide than the c16-AHL 3 K 3 -CO 2 H peptide, it is of interest to quantitatively determine how much of the titanium precursor is consumed by the peptide. This was achieved by a twofold approach, (1) analyse the turbidity of the sample with respect to increasing TiBALDH concentration and (2) use a colorimetric assay in which 3,4 dihydroxybenzoic acid (dhba) is used to coordinate with the remaining TiBALDH in solution generating [Ti(dhba) 3 ] 2− , λ max =380 nm (refs 18 , 32 , 33 ). As discussed, the peptides in water do not assemble into any observable structure. When performing the titrations under unassembled conditions, we found that c16-AHL 3 K 3 -CO 2 H and c16-AHL 3 K 9 -CO 2 H consumed 19±1 and 38±2 molar equivalents of the TiBALDH precursor respectively, see Supplementary Figs 7,8 . This was not surprising due to the simple fact that more lysines are present on the longer peptide. Analysing the peptides under assembled conditions we found that c16-AHL 3 K 9 -CO 2 H was found to convert the same molar equivalents of TiBALDH to TiO 2 as the unassembled structure, 38±2 mol. eq. (see Supplementary Fig. 8 ), whereas the assembled c16-AHL 3 K 3 -CO 2 H was found to consume more than twofold fewer titanium equivalents, 7±1 mol. eq. (see Supplementary Fig. 7 ) than the analogous unassembled study. This can be explained by the high degree of bundling in the sample resulting in fewer displayed lysine residues available for mineralization. Consistent with the electron microscopy studies, we find that the unbundled peptide fibres of c16-AHL 3 K 9 -CO 2 H yield an efficient TiO 2 mineralization platform whereas the heavily bundled structure of c16-AHL 3 K 3 -CO 2 H yields fewer TiO 2 nanoparticles due to the loss of exposed lysine. The two materials generated provide an excellent platform for comparing efficient electron transfer between the metalloporphyrin dye and the nanoparticulate semiconducting TiO 2 . Dye incorporation We previously reported the ability to incorporate zinc protoporphyrin IX ((PPIX)Zn) into the assembled peptide amphiphile, c16-AHL 3 K 3 -CO 2 H [15] . In the present study, we replaced (PPIX)Zn with (DPP)Zn. (PPIX)Zn was found to be sensitive to room light and would decompose in less than 24 h. With this knowledge, the porphyrin (DPP)Zn replaced the (PPIX)Zn molecule. This non-natural molecule was intentionally chosen because it serves as a basic building block in more complex porphine systems that have a wide array of functionalities and applications such as: nonlinear optics, molecular beacons, biomolecular imaging reagents and light-harvesting antennae [34] , [35] , [36] , [37] , [38] , [39] . To incorporate the (DPP)Zn dye molecule, a 125 μM peptide solution was aged for 15 min in 100 mM NH 4 OH at 65 °C before addition of (DPP)Zn, 25 μM. Due to the increased hydrophobicity of the (DPP)Zn in comparison with the (PPIX)Zn molecule, it was necessary to heat the samples to >80 °C followed by sonication to achieve successful chromophore incorporation. We verified the presence of the axially coordinated zinc porphyrin complex by ultraviolet (UV)/visible spectroscopy, Fig. 5 . In the absence of peptide following the above sample preparation, (DPP)Zn in 100 mM NH 4 OH yields a very broad spectrum: split B-band ( λ max =415, 476 nm) and Q-band ( λ max =558, 590 nm). A broad red-shifted spectrum signifies aggregation [40] , [41] , [42] . (DPP)Zn (25 μM) in the presence of the assembled c16-AHL 3 K 3 -CO 2 H and c16-AHL 3 K 9 -CO 2 H (125 μM) in 100 mM NH 4 OH yields a sharp spectrum typical of histidyl axial coordination B-band ( λ max =426 nm) and Q-bands ( λ max =554, 592 nm). Circular dichroism spectroscopy confirms the maintenance of the exciton coupling between neighbouring chromophores as shown by the intense Cotton effect ( λ max =423 nm, λ min =416 nm) similar to our previous report [15] . Furthermore, the maintenance of the supramolecular morphology in the presence of the dye was analysed and confirmed to be similar to that found in the absence of (DPP)Zn, see Supplementary Figs 2,3 . At this point, TiBALDH was added to the pre-assembled fibres to total 1 wt% in solution. Mineralization on the surface of the peptide occurred for 10 min at 65 °C. The sample was pelleted via centrifugation and resuspended in fresh solvent three times to remove excess TiBALDH. We find very little change in the visible spectrum with the exception of a slight increase in baseline absorptivity due to scattering from the increased turbidity of the solution. In the CD spectrum, this leads to a slight decrease in the intensity. Also, the electron microscopy indicates that the addition of the metalloporphyrin does not disrupt the fibril structure including when TiO 2 is mineralized on the peptide surface, Fig. 3c,f . Thus, a platform for charge separation events similar to that of DSCs is generated, in which the orientation and spatial distance between the dye and the inorganic material is well controlled and structurally predictable. 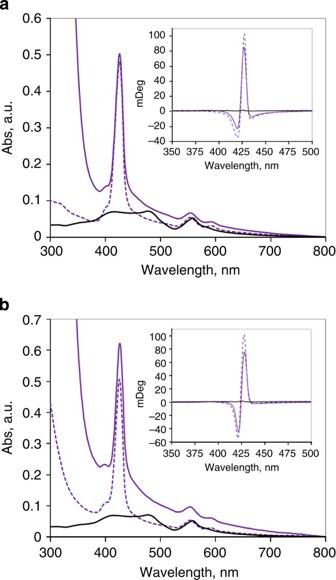Figure 5: Incorporation of the dye molecule, (DPP)Zn, into the assembled peptide amphiphile. (a) UV/visible spectra of (DPP)Zn (black line), (DPP)Zn:c16-AHL3K3-CO2H (dashed purple line), and (DPP)Zn:c16-AHL3K3-CO2H:TiO2(solid purple line). All samples are in 100 mM NH4OH. Inset: Circular dichroism spectra of (DPP)Zn (black line), (DPP)Zn:c16-AHL3K3-CO2H (dashed purple line) and (DPP)Zn:c16-AHL3K3-CO2H:TiO2(solid purple line). (b) Analagous spectra toafor (DPP)Zn:c16-AHL3K9-CO2H. Abs, absorbance. Figure 5: Incorporation of the dye molecule, (DPP)Zn, into the assembled peptide amphiphile. ( a ) UV/visible spectra of (DPP)Zn (black line), (DPP)Zn:c16-AHL 3 K 3 -CO 2 H (dashed purple line), and (DPP)Zn:c16-AHL 3 K 3 -CO 2 H:TiO 2 (solid purple line). All samples are in 100 mM NH 4 OH. Inset: Circular dichroism spectra of (DPP)Zn (black line), (DPP)Zn:c16-AHL 3 K 3 -CO 2 H (dashed purple line) and (DPP)Zn:c16-AHL 3 K 3 -CO 2 H:TiO 2 (solid purple line). ( b ) Analagous spectra to a for (DPP)Zn:c16-AHL 3 K 9 -CO 2 H. Abs, absorbance. Full size image Charge-separated state The characterized self-assembled hybrid material, c16-AHL 3 K 9 -CO 2 H:(DPP)Zn:TiO 2 , yields a platform in which the external semiconducting TiO 2 and the internal dye molecule, (DPP)Zn, are separated by a specific distance determined by the length of the peptide chain. Here, we presume that the three leucine residues separate the dye molecule, which is axially coordinated to the histidine residue, and the TiO 2 , which is mineralized by the lysine residues, Fig. 2 . The distance from the histidine to the first lysine residue is >13 Å along the peptide backbone. To spectroscopically observe a photoinduced charge-separated state, electron paramagnetic resonance (X-band, 9.4 GHz) was employed to observe the characteristic signatures of the electron/hole pair of the zinc porphyrin cation radical and lattice-trapped electrons within TiO 2 . Three samples were analysed under visible illumination ( λ >400 nm) to confirm the charge-separated state: (1) c16-AHL 3 K 9 -CO 2 H:TiO 2 , (2) c16-AHL 3 K 9 -CO 2 H:(DPP)Zn and (3) c16-AHL 3 K 9 -CO 2 H:(DPP)Zn:TiO 2 . In sample (1), no signal was observed as expected under visible illumination. However, when illuminating with UV/visible light we observe a signature spectrum for reduced anatase titania [43] and an oxidized species ( g =2.004), presumably a -CH radical on the peptide as characterized by the presence of a doublet with a 17 G hyperfine coupling, see Supplementary Fig. 9 (ref. 44 ). The observation of anatase TiO 2 confirms our findings in the HRTEM studies ( vide infra). In sample (2), we observe a single line at g =2.004. Somewhat surprisingly, a triplet species of excited (DPP)Zn is not observed. Our previous report suggests that a triplet species is never formed due to an exciton annihilation mechanism [15] . Here, the observed spectrum is typical of a zinc porphyrin cation radical, but no acceptor moiety is present. It is also possible that charge separation along the axis of the assembled porphyrins is occurring in which a separated cation radical (DPP)Zn + and an anion radical (DPP)Zn − result [45] . Both species have a similar g value of ~2.004 and vary only in line width, which would yield a spectrum consistent with that observed in sample (2). It is prudent to note that in the absence of the peptide, (DPP)Zn yields a typical triplet spectrum as has been seen in related molecules, see Supplementary Fig. 10 (refs 46 , 47 ). Finally, in sample (3) we observe a signal from the cation radical of (DPP)Zn dye ( g =2.003) and the signal that corresponds to anatase lattice trapped electrons ( g ⊥ =1.990, g || 1 =1.961 and g || 2 =1.958) (ref. 43 ). 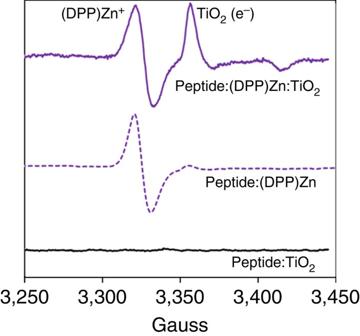Figure 6: Charge separation in the hybrid peptide/(DPP)Zn/TiO2structure. X-band EPR spectra of c16-AHL3K9-CO2H:TiO2(black line), c16-AHL3K9-CO2H:(DPP)Zn (purple dotted line) and c16-AHL3K9-CO2H:(DPP)Zn:TiO2(purple line) frozen in 100 mM NH4OH at 10 K and illuminated with visible light (>400 nm). Figure 6 illustrates the observed phenomenon, in which the dye molecule, excited by visible light, transfers an electron to the nanocrystalline anatase TiO 2 . Charge recombination was not observed at low temperatures (up to 20 K) but upon warming the sample to RT and then cooling back down to 20 K, all signals were absent indicating that complete charge recombination had occurred during the thaw–freeze process. Figure 6: Charge separation in the hybrid peptide/(DPP)Zn/TiO 2 structure. X-band EPR spectra of c16-AHL 3 K 9 -CO 2 H:TiO 2 (black line), c16-AHL 3 K 9 -CO 2 H:(DPP)Zn (purple dotted line) and c16-AHL 3 K 9 -CO 2 H:(DPP)Zn:TiO 2 (purple line) frozen in 100 mM NH 4 OH at 10 K and illuminated with visible light (>400 nm). Full size image The peptide sequence is also important in tuning the efficient transfer of electrons from the excited (DPP)Zn molecule to the TiO 2 particles. Here, we comparatively analysed the samples c16-AHL 3 K 3 -CO 2 H:(DPP)Zn:TiO 2 and c16-AHL 3 K 9 -CO 2 H:(DPP)Zn:TiO 2 . We found that more lysine residues result in more TiO 2 on the surface of the assembled peptide. When we analyse these two samples by X-band electron paramagnetic resonance (EPR), we find that indeed more lysine amino acids/more TiO 2 results in more electrons injected into TiO 2 . Specifically, when c16-AHL 3 K 3 -CO 2 H:(DPP)Zn:TiO 2 is illuminated with visible light, we see the same signal from the (DPP)Zn cation radical but the signal from the lattice-trapped electrons in TiO 2 is significantly diminished when compared with that of c16-AHL 3 K 9 -CO 2 H, see Supplementary Fig. 11 . While these results were expected, they highlight the degree to which these materials can be tailored through peptide sequence variation. In summary, we have developed a new material inspired by the photoinitiated redox pathways in nature in which a peptide amphiphile capable of binding a metalloporphyrin for solar harvesting can also mineralize TiO 2 on the surface of the peptide yielding a nanostructured, organic/inorganic hybrid material. We were able to confirm the simple notion that increasing the number of positively charged lysine residues leads to more mineralization of TiO 2 on the peptide surface. This could also be explained by the larger exposed surface area in the less-bundled c16-AHL 3 K 9 -CO 2 H assembly. Electron microscopy studies show that both peptides are decorated with anatase TiO 2 where the metal oxide is specifically associated with the peptide fibres. Furthermore, we successfully mineralized TiO 2 on the assembled peptide structure when the dye molecule (DPP)Zn was axially coordinated to an imidazole nitrogen of the histidine residue generating a platform for executing charge separation studies. Upon illumination of this complex hybrid material, electron paramagnetic resonance clearly indicated a charge-separated state between the coordinated (DPP)Zn and the mineralized TiO 2 yielding a (DPP)Zn + /TiO 2 (e − ) hole/electron pair. The degree of charge separation can be modulated through variations in the peptide sequence. In particular, increasing the number of lysine residues that are responsible for mineralization yields more TiO 2 and therefore an increased number of charge-separated states. This simple peptide design that affords a complex material will allow us to explore the ability to tune the material through variations in peptide sequence, porphyrin selection, porphyrin position and added redox hopping sites to tune the electron transfer pathway rate and efficiency. The observed charge separation will also allow us to explore the assembly as the fundamental construct of DSCs [5] , [6] and photocatalytic water-splitting systems [48] , [49] . Peptide and porphyrin synthesis The synthetic procedure for c16-AHL 3 K 3 -CO 2 H has been reported in our previous studies. The synthesis of c16-AHL 3 K 9 -CO 2 H, cleavage from the resin and purification followed the same strategy as the previously reported peptide with the addition of six lysine residues in the sequence. Matrix-assisted laser desorption/ionization–time of flight mass spectrometry was used to identify the peptide; calculated for C 97 H 185 N 25 O 16 +H + , 1957.45 m/z ; found, 1957.25 m/z . The synthetic procedures for (DPP)Zn are well known following the Lindsey condensation method using trifluoroacetic acid as a catalyst and dichlorodicyanobenzoquinone to complete ring oxidation [50] . The full synthesis of (DPP)Zn is outlined in Supplementary Fig. 12 . Peptide assembly Solutions of the peptide amphiphiles (500 μM) were made by dilutions from a concentrated stock solution in water (c16-AHL 3 K 3 -CO 2 H, 1 wt%, 8.4 mM or c16-AHL 3 K 9 -CO 2 H, 1 wt%, 5.1 mM) with either water (Millipore) or ammonium hydroxide (NH 4 OH, 100 mM). The samples were heated to 65 °C for 15 min to ensure complete β-sheet formation and assembly. Thermal folding measurements were performed by monitoring the n-π* transitions at 210 and 223 nm of the circular dichroism (JASCO J-815) spectra from 10–65 °C. Spectra were monitored at 20 °C. Metalloporphyrin binding To incorporate the metalloporphyrin moiety to the assembled peptide, 1.5 μl of a (DPP)Zn stock solution (10 mM in dimethylsulphoxide) was added to a 600 μl solution of assembled peptide to yield a 25 μM final concentration. Due to the hydrophobic nature of (DPP)Zn, the solution was heated to >80 °C for 15 min and sonicated briefly (<10 s) before returning to the hot bath. This process is repeated three times. Circular dichroism spectroscopy was used to monitor the exciton coupling intensity to follow the binding event and UV/visible spectroscopy (Cary 50 Spectrophotometer) was used to confirm that the binding event was complete. Upon completion of binding, the sample was cooled to RT and rested for 1 h. Mineralization studies TiBALDH (Sigma-Aldrich, 50 wt% in water) was used as a water soluble precursor to TiO 2 . The concentration of TiBALDH was varied with respect to peptide concentration to determine how much TiO 2 was being formed on the surface of the peptide. We observed TiO 2 formation by employing two methods. First, we monitored the turbidity of the solution by UV/visible spectroscopy. Briefly, 300 μl of a 500 μM solution of the peptide amphiphile (without (DPP)Zn) in either water or 100 mM NH 4 OH was placed in a quartz cuvette ( l =1.0 mM). From a TiBALDH stock solution in water (150 mM) 1.0 μl aliquots were added resulting in 0.5 mM addition of TiBALDH added per aliquot. The samples were heated to 65 °C for 10 min to ensure reaction completion. A total of 20.0 μl of TiBALDH stock solution were added to complete the study. Secondly, a colourimetric assay was employed to support the turbidity data. Similar to the TIRON assay [18] , [32] , [33] , we centrifuged the samples to pellet the material. When the clear supernatant containing unreacted TiBALDH is mixed with an excess of dhba (or similar catechol), the molecule [Ti(dhba) 3 ] 2− results which yields a yellow-orange solution, λ max =380 nm ( ε =3,345 M −1 cm −1 ). As a result, the amount of consumed TiBALDH precursor can be determined. When preparing samples for microscopy analysis, 300 μl of a 500 μM solution of the peptide amphiphile in either water or 100 mM NH 4 OH was placed in an Eppendorf tube. TiBALDH, 6 μl of a 50 wt% stock, was added to the sample resulting in a final 1 wt% or 35 mM TiBALDH concentration. The sample was incubated at 65 °C for 10 min. Following incubation, the samples were centrifuged (10 g for 2 min) yielding a clear-to-white pellet depending on the peptide. The supernatant was removed via pipetting followed by pellet resuspension with fresh water or 100 mM NH 4 OH (300 μl). Sample washing was repeated three times. Electron microscopy Seven microlitres of the samples were drop cast onto a 400 mesh copper grid with a carbon or Holey carbon support film (Ted Pella). After 2 min, the excess solution was wicked away and the sample dried under ambient conditions. Analysis of the self-assembled peptide with and without TiO 2 mineralized on its surface was analysed by scanning electron microscopy with a transmission detector (JEOL 7500 FE-SEM). Confirmation of successful mineralization of TiO 2 was analysed by energy dispersive X-ray spectroscopy. When more detailed analysis of the system was required, the samples were analysed with transmission electron microscopy (JEOL JEM-2010F). HRTEM and EFTEM were used to analyse the crystalline nature of the TiO 2 and map out the distribution of the TiO 2 , respectively. Furthermore, electron diffraction analysis enabled the determination of the crystal phase formed. Electron paramagnetic resonance Samples for EPR were concentrated to 2 mM (DPP)Zn and 10 mM Peptide in 100 mM NH 4 OH. X-band continuous wave EPR experiments were carried out using a Bruker ELEXSYS E580 spectrometer operating in the X-band (9.4 GHz) and equipped with an Oxford CF935 helium flow cryostat with an ITC-5025 temperature controller. A 300 W Xe UV lamp (ILC) with 400 nm cutoff and water as IR filters was used as the light source. The g factors were calibrated for homogeneity and accuracy by comparison with a coal standard, g =2.00285±0.00005. The samples were deaerated, equilibrated in a nitrogen atmosphere for a minimum of 30 min before EPR measurement. How to cite this article: Fry, H. C. et al . Photoinitated charge separation in a hybrid titanium dioxide metalloporphyrin peptide material. Nat. Commun. 5:4606 doi: 10.1038/ncomms5606 (2014).